Scara1deficiency impairs clearance of soluble amyloid-β by mononuclear phagocytes and accelerates Alzheimer’s-like disease progression In Alzheimer’s disease, soluble amyloid-β causes synaptic dysfunction and neuronal loss. Receptors involved in clearance of soluble amyloid-β are not known. Here we use short hairpin RNA screening and identify the scavenger receptor Scara1 as a receptor for soluble amyloid-β expressed on myeloid cells. To determine the role of Scara1 in clearance of soluble amyloid-β in vivo , we cross Scara1 null mice with PS1-APP mice, a mouse model of Alzheimer’s disease, and generate PS1-APP- Scara1- deficient mice. Scara1 deficiency markedly accelerates Aβ accumulation, leading to increased mortality. In contrast, pharmacological upregulation of Scara1 expression on mononuclear phagocytes increases Aβ clearance. This approach is a potential treatment strategy for Alzheimer’s disease. Work in transgenic mouse models of Alzheimer’s disease (AD) indicates that mononuclear phagocytes can promote the clearance of amyloid-β (Aβ) peptides. Reduction in the number of recruited mononuclear phagocyte led to accelerated Aβ deposition especially around blood vessels, leading to intracerebral haemorrhage and increased mortality in a mouse model of AD [1] . In support of these findings, depletion of perivascular macrophages significantly increased the number of Thioflavin S-positive cortical blood vessels and total perivascular Aβ levels [2] . Conversely, stimulation of perivascular macrophage turnover or enhancing recruitment of peripheral monocytes reduced cerebral perivascular and parenchymal Aβ load [2] , [3] . These data suggest that mononuclear phagocytes may delay progression of AD by promoting clearance of Aβ and preventing senile plaque formation. However, persistent Aβ accumulation in spite of increasing mononuclear phagocyte numbers in AD suggests that the ability of these cells to clear Aβ may decrease with age and progression of AD pathology [4] . Much attention has been focused for many years on the insoluble aggregates of Aβ found in senile plaques. Insoluble fibrillar aggregates are neurotoxic in vitro and activate microglia and astrocytes to produce cytokines, chemokines and reactive oxygen and nitrogen species [5] , however, the number of senile plaques in any particular areas of the brain does not always correlate with neuronal death or synaptic loss in that area [6] , [7] , [8] . Such discrepancy brought attention to other non-aggregated forms of Aβ [9] , [10] . These soluble Aβs (sAβs) include Aβ monomers or oligomers that remain soluble in aqueous buffers after high-speed ultracentrifugation [9] , [10] . sAβ may start accumulating in the brain before formation of visible senile plaques. sAβ is associated with cognitive dysfunction in transgenic mice, and several groups confirmed that a strong correlation exists between sAβ levels and synaptic loss and neuronal degeneration [6] , [7] , [8] , [9] , [10] , [11] , [12] . It is not known whether sAβ interacts with monocytes, microglia or the potential receptors involved in such interactions. However, because sAβ starts accumulating before formation of senile plaques and microglia are constantly surveying their environment for any potential injurious stimuli [13] , we hypothesized that mononuclear phagocytes can recognize and bind sAβ. Microglia and macrophages express several receptors that can promote binding and/or phagocytosis of fibrillar Aβ aggregates in vitro . These include the class A1 scavenger receptors ( Scara1 ) [14] , the class B2 scavenger receptors ( Scarb2 ) or CD36 (refs 5 , 15 ), RAGE [16] and others. Mononuclear phagocytes also express a number of Aβ-degrading enzymes, such as insulysin, neprilysin and others [4] , [17] . The exact role of each of these receptors in development or progression of AD is not known. We found that as transgenic AD mice age, expression of these Aβ phagocytic receptors and Aβ-degrading enzymes decreased significantly in microglia, thereby promoting Aβ accumulation and contributing to neurodegeneration [4] . This led us to hypothesize that restoring the ability of mononuclear phagocytes to phagocytose or degrade Aβ may be a therapeutic modality to delay or stop the progression of AD. In support of this hypothesis, genetic downregulation of the transforming growth factor-β-Smad2/3 innate immune signalling pathway, led to increased infiltration of macrophages around blood vessels, and decreased Aβ levels and behavioural deficits in AD mice [3] . It is not known if pharmacological stimulation of the mononuclear phagocyte Aβ clearance pathways will also lead to mitigation of AD-like pathology. In this paper, we use a short hairpin RNA (shRNA) screen to identify receptors for sAβ and show that Scara1 is a phagocytic receptor that mediates clearance of sAβ in vitro , and that Scara1 deficiency is associated with increased early mortality and Aβ deposition in the PS1-APP mouse model of AD. We also show that pharmacological upregulation of Scara1 leads to increased Aβ clearance, suggesting that this approach may be a strategy for treatment of AD. shRNA screen identifies Scara1 as a receptor for sAβ uptake To identify mononuclear phagocyte receptors involved in the uptake of sAβ, we used a mouse shRNA library targeting innate immune receptors to screen for genes that mediate macrophage uptake of sAβ labelled with the fluorescent dye Hilyte-Fluor 488. We confirmed that our Hilyte-Fluor 488 Aβ is soluble using native electrophoresis and Thioflavin S staining ( Supplementary Fig. S1a,b ) as described [5] , [6] , [7] , [8] . The RNAi Consortium has previously published that its lentiviral library silences genes in a diverse set of cell types, contains five shRNA for nearly every gene in the murine genome, and is capable of significantly reducing target mRNA levels ( Fig. 1a ) [18] . Using a subset of the mouse lentiviral shRNA library targeting toll-like receptors, scavenger receptors and other pattern-recognition receptors [19] , we performed a screen to identify genes that mediate macrophage uptake of sAβ 1–42 Hilyte-Fluor 488 using RAW 264.7 (RAW) macrophages. Silencing expression of all receptors tested was effectively performed to ~20% of normal expression ( Fig. 1a , data not shown). Interestingly, only silencing of the scavenger receptors CD36 and Scara1 led to a significant reduction in sAβ 1–42 Hilyte-Fluor 488 uptake by RAW macrophages ( Fig. 1b , data not shown). The results of our shRNA screen indicate that Scara1 and CD36 can mediate uptake of sAβ by mononuclear phagocytes in vitro . Gene silencing of other scavenger receptors, such as Scarb1 , Scarf , CD68 and CXCL16 also expressed by macrophages, had no effect on uptake of sAβ 1–42 Hilyte-Fluor 488 by RAW cells ( Fig. 1b ), suggesting that Scara1 and CD36 are the main receptors involved in this process. 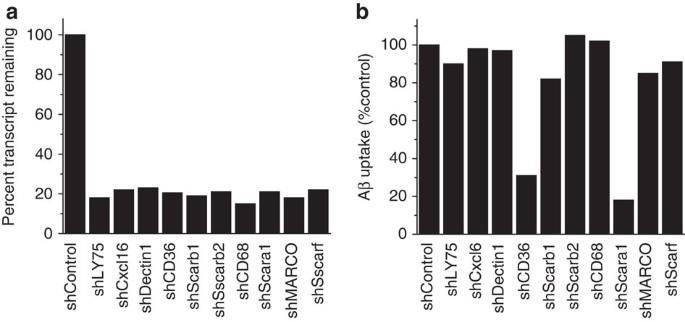Figure 1: A shRNA screen identifiesScara1as a receptor for sAβ. (a) RAW macrophages were transduced with lentivirus encoding gene-specific shRNAs to 30 pattern-recognition receptors or with a control shRNA directed against green fluorescent protein. Gene expression was measured by qPCR, and 3–5 individual shRNAs per gene were identified that significantly reduced mRNA expression. (b) Pattern-recognition receptor expression was knocked down in individual pools of RAW macrophages, which were then incubated with Hilyte-Fluor 488-labelled sAβ 1–42 for 2 h. Cell-associated sAβ was then quantified by flow cytometry. Data are from a representative experiments repeated three times with similar results. Figure 1: A shRNA screen identifies Scara1 as a receptor for sAβ. ( a ) RAW macrophages were transduced with lentivirus encoding gene-specific shRNAs to 30 pattern-recognition receptors or with a control shRNA directed against green fluorescent protein. Gene expression was measured by qPCR, and 3–5 individual shRNAs per gene were identified that significantly reduced mRNA expression. ( b ) Pattern-recognition receptor expression was knocked down in individual pools of RAW macrophages, which were then incubated with Hilyte-Fluor 488-labelled sAβ 1–42 for 2 h. Cell-associated sAβ was then quantified by flow cytometry. Data are from a representative experiments repeated three times with similar results. Full size image To confirm that uptake of sAβ by microglia is indeed a receptor-mediated event, we incubated N9 microglia with increasing concentrations of sAβ and quantified uptake by flow cytometry. As seen in Fig. 2a , uptake of sAβ by microglia began to reach saturation at ~2 μM. In addition, uptake of sAβ by N9 microglia was time dependent and reached saturation at ~4 h ( Fig. 2b ). These data indicate that uptake of sAβ by microglia is likely to be receptor-mediated and is saturable in a dose- and time-dependent manner. To further confirm that uptake of sAβ by microglia is mediated by scavenger receptors, we incubated N9 cells for 2 h with 1 μM sAβ 1–42 Hilyte-Fluor 488±200 μM Fucoidan, a broad inhibitor of scavenger receptors, and measured uptake by flow cytometry. Fucoidan significantly inhibited the amount of sAβ taken by N9 microglia ( Fig. 2c ) and the number of cells that took sAβ ( Fig. 2d ). 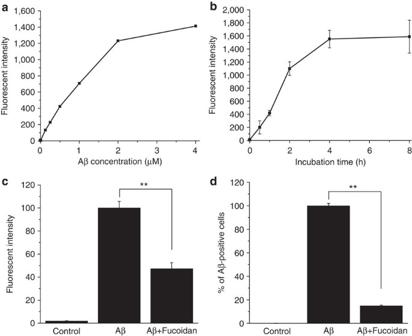Figure 2: Uptake of sAβ by N9 microglia. (a,b) Uptake of Hilyte-Fluor 488-labelled sAβ by N9 microglia is saturable in a dose- and time-dependent manner. (c,d) N9 cells were pretreated with 200 μg ml−1Fucoidan, a broad inhibitor of scavenger receptors, and then incubated with 1 μM freshly dissolved Hilyte-Fluor 488-labelled sAβ 1–42 for 2 h. The uptake of sAβ was measured by flow cytometry. Fucoidan significantly inhibited the amount of sAβ taken up by N9 cells and the number of cells that took sAβ, indicating that microglial scavenger receptors are essential for phagocytosis of soluble Aβ. Values are mean±s.e.m.n=3 (analysis of variance, **P<0.05). Figure 2: Uptake of sAβ by N9 microglia. ( a , b ) Uptake of Hilyte-Fluor 488-labelled sAβ by N9 microglia is saturable in a dose- and time-dependent manner. ( c , d ) N9 cells were pretreated with 200 μg ml −1 Fucoidan, a broad inhibitor of scavenger receptors, and then incubated with 1 μM freshly dissolved Hilyte-Fluor 488-labelled sAβ 1–42 for 2 h. The uptake of sAβ was measured by flow cytometry. Fucoidan significantly inhibited the amount of sAβ taken up by N9 cells and the number of cells that took sAβ, indicating that microglial scavenger receptors are essential for phagocytosis of soluble Aβ. Values are mean±s.e.m. n =3 (analysis of variance, ** P <0.05). Full size image Scara1 deficiency is associated with reduced sAβ uptake Expression of Scara1 in HEK293 cells is sufficient to promote the ability of these cells to take Aβ ( Supplementary Fig. S2 ). To determine if Scara1 is necessary for uptake of sAβ by primary monocytes and microglia as suggested by our shRNA screen in macrophages, we isolated circulating monocytes and microglia from adult mice with targeted deletion of various scavenger receptors and from wild-type (WT) mice and tested the ability of these freshly isolated monocytes and microglia to take up sAβ. Interestingly, only targeted deletion of Scara1 led to a significant reduction in the uptake of sAβ by fresh monocytes ( Fig. 3a ) and microglia ( Fig. 3b ) by 65% and 50%, respectively. Targeted deletion of CD36 did not affect uptake of sAβ by monocytes and only reduced its binding to microglia by 25%, which was not statistically significant. These data indicate that Scara1 is a major receptor for uptake of sAβ by monocytes and microglia and that Scara1 -mediated uptake is not redundant. The lack of effect of targeted deletion of CD36 on sAβ uptake suggests that unlike Scara1 , CD36 does not have a non-redundant role in clearance of sAβ. Because targeted deletion of CD36 leads to reduced Aβ-induced activation of mononuclear phagocytes to produce cytokines and reactive oxygen species, our data suggest that CD36 may be involved in the activation of mononuclear phagocytes by sAβ and not in the clearance of sAβ by these cells [5] , [20] , [21] . This is reminiscent of the role that CD36 has in the interaction between macrophages and oxidized low-density lipoproteins (LDLs) [22] . 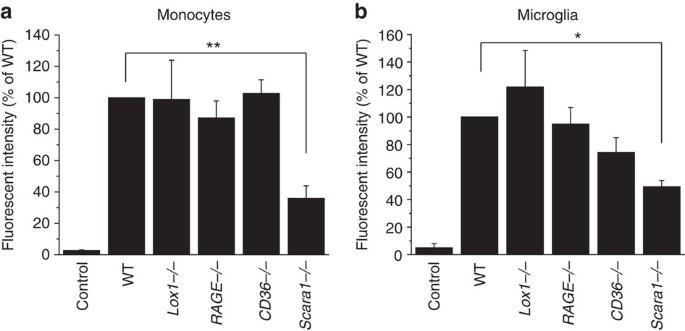Figure 3: Scara1 is a major monocyte and microglial receptor for sAβ. Targeted deletion ofScara1, but notCD36,LOX-1orRAGE, significantly reduces sAβ uptake by CD11b+ monocytes (a) and microglia (b). Monocytes and microglia isolated from C57BL6 mice or mice with targeted deletion of the indicated gene were incubated with 1 μM Hilyte-Fluor 488-labelled sAβ 1–42 for 2 h, and uptake of sAβ was measured by flow cytometry. Data points represent the mean of triplicate determinations±s.e.m.,n=4 (analysis of variance, *P<0.05, **P<0.03). Figure 3: Scara1 is a major monocyte and microglial receptor for sAβ. Targeted deletion of Scara1 , but not CD36 , LOX-1 or RAGE , significantly reduces sAβ uptake by CD11b+ monocytes ( a ) and microglia ( b ). Monocytes and microglia isolated from C57BL6 mice or mice with targeted deletion of the indicated gene were incubated with 1 μM Hilyte-Fluor 488-labelled sAβ 1–42 for 2 h, and uptake of sAβ was measured by flow cytometry. Data points represent the mean of triplicate determinations±s.e.m., n =4 (analysis of variance, * P <0.05, ** P <0.03). Full size image Increased mortality in PS1-APP- Scara1 −/− mice To determine if Scara1 mediates clearance of sAβ in vivo , and the effects of such clearance on accumulation of Aβ, we generated PS1-APP- Scara1 − / − mice and analysed these mice for Aβ levels and AD-like pathology. To accomplish this, we utilized a strategy that we have successfully used in the past to generate transgenic APP mice deficient in the chemokine receptor Ccr2 (ref 1 ). Briefly, PS1-APP mice on a C57BL6 background were crossed to Scara1 −/− mice (also on a C57BL6 background) to generate PS1-APP- Scara1 +/ − mice. We then crossed these mice with Scara1 −/− mice to generate PS1-APP- Scara1 − / − mice. PS1-APP- Scara1 +/ − and PS1-APP- Scara1 − / − mice initially appeared healthy, without obvious behavioural abnormalities. However, after reaching 7 weeks of age, there was a marked increase in the mortality rate of both PS1-APP- Scara1 +/ − and PS1-APP- Scara1 − / − mice as compared with control PS1-APP mice ( Fig. 4a ). By the age of 160 days, 39% of PS1-APP- Scara1 − /+ and 53% of PS1-APP- Scara1 − / − mice had died, compared with 16% of PS1-APP mice. The number of dying PS1-APP- Scara1 +/ − mice reached a plateau at age 108 days, whereas PS1-APP- Scara1 − / − mice continued to die until our data collection had stopped by age 160 days. And while PS1-APP- Scara1 − / − mice had higher mortality at 160 days than PS1-APP- Scara1 +/ − mice, the overall difference between those two genotypes did not reach statistical significance ( Fig. 4a ). These data show that Scara1 deficiency leads to increased mortality in mice expressing the PS1-APP transgenes. These data are similar to what we found with Ccr2 deficiency (a defect that leads to reduced mononuclear phagocyte recruitment but does not affect their function [1] ). These data indicate that blocking mononuclear phagocyte number or function has detrimental effect in AD mouse models. 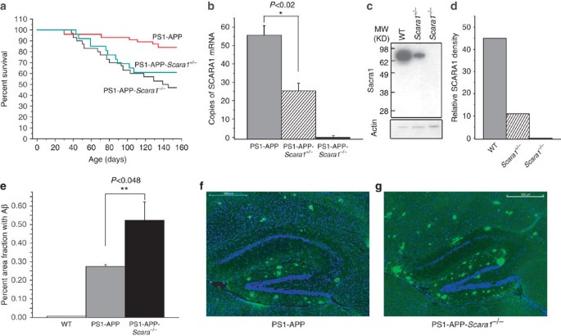Figure 4:Scara1deficiency is associated with increased mortality and higher Aβ deposition in PS1-APP mice. (a) Survival curves for PS1-APP (n=30), PS1-APP-Scara1−/+(n=25) and PS1-APP-Scara1−/−(n=24) mice. (b) Level ofScara1mRNA in PS1-APP-Scara1+/−mice is 45% that of PS1-APP mice. Reduced gene dosage inScara1+/−miceis associated with a 76% reduction inScara1protein levels as shown in this representative western blot (c) and quantified by densitometry (d); representative blot and quantification were repeated three different times with similar results. (e–g)Scara1deficiency significantly increases Aβ deposition in 8-month-old PS1-APP mice. Increased number of visible Aβ deposits in PS1-APP-Scara1−/−brains (g) compared with PS1-APP brains (f). Scale bars, 500 μm. Data points represent the average of five independent determinations per mouse,±s.e.m.,n=4–6 mice per group (analysis of variance, *P<0.02, **P<0.048). Figure 4: Scara1 deficiency is associated with increased mortality and higher Aβ deposition in PS1-APP mice. ( a ) Survival curves for PS1-APP ( n =30), PS1-APP- Scara1 − /+ ( n =25) and PS1-APP- Scara1 − / − ( n =24) mice. ( b ) Level of Scara1 mRNA in PS1-APP- Scara1 +/ − mice is 45% that of PS1-APP mice. Reduced gene dosage in Scara1 +/− mice is associated with a 76% reduction in Scara1 protein levels as shown in this representative western blot ( c ) and quantified by densitometry ( d ); representative blot and quantification were repeated three different times with similar results. ( e – g ) Scara1 deficiency significantly increases Aβ deposition in 8-month-old PS1-APP mice. Increased number of visible Aβ deposits in PS1-APP- Scara1 − / − brains ( g ) compared with PS1-APP brains ( f ). Scale bars, 500 μm. Data points represent the average of five independent determinations per mouse,±s.e.m., n =4–6 mice per group (analysis of variance, * P <0.02, ** P <0.048). Full size image As expected, Scara1 mRNA levels in the brains of PS1-APP- Scara1 +/ − mice were ~45% of those in PS1-APP mice and were not detectable in PS1-APP- Scara1 −/− mice as determined by quantitative real-time PCR (qPCR) ( Fig. 4b ). A similar trend was observed in WT, Scara1 +/− and Scara1 −/− mice (not shown). Interestingly, analysis of Scara1 protein expression by western blot showed that 55% reduction in Scara1 gene dosage (as occurs in Scara1 +/ − mice) is associated with a much larger 76% reduction in Scara1 protein level ( Fig. 4 c ). Because survival of PS1-APP mice appears to correlate with Scara1 expression, it is possible that efficient clearance of Aβ requires a certain threshold of Scara1 expression, and the disproportionate reduction in Scara1 protein levels in Scara1 +/ − mice, likely below such threshold, may explain the comparable mortality rates between PS1-APP- Scara1 +/ − and PS1-APP- Scara1 − / − mice. Increased Aβ accumulation in PS1-APP- Scara1 −/− mice To determine the effects of Scara1 deficiency on AD-like pathology, we analysed the brains of 8-month-old PS1-APP- Scara1 − / − mice for Aβ deposition in comparison with PS1-APP mice. As seen in Fig. 4e–g , Scara1 deficiency led to a significant increase in the surface area fraction of the brain stained for Aβ in PS1-APP mice. As expected, WT mice did not have any Aβ in their brain at this age ( Fig. 2e ). These data support the results obtained from our shRNA screen and from the experiments showing decreased uptake of sAβ in vitro by monocytes and microglia isolated from Scara1 − / − mice ( Fig. 3a ). The data further indicate that Scara1 is a major receptor involved in endogenous clearance of Aβ and that deficiency in Scara1 , as occurs in aging AD mice [4] , is associated with increased Aβ levels. Our shRNA-screening data showed that CD36 can mediate uptake of sAβ. RAGE has been also shown to be a receptor for Aβ [16] . To determine if Scara1 deficiency indirectly affected CD36 or RAGE expression, we measured CD36 and RAGE mRNA in young (150 days) WT, Scara1 −/− , PS1-APP and PS1-APP- Scara1 − / − brains by qPCR. As seen in Fig. 5a , Scara1 deficiency did not affect CD36 mRNA levels in Scara1 − / − or PS1-APP- Scara1 − / − brains. Furthermore, we did not detect any difference in expression of RAGE in PS1-APP- Scara1 − / − mice compared with PS1-APP mice (Not shown). These data indicate that increased Aβ deposition in PS1-APP- Scara1 − / − brains is likely due to decreased Scara1 -mediated Aβ clearance in these mice and not due to a change in expression of other Aβ receptors such as Cd36 and RAGE. 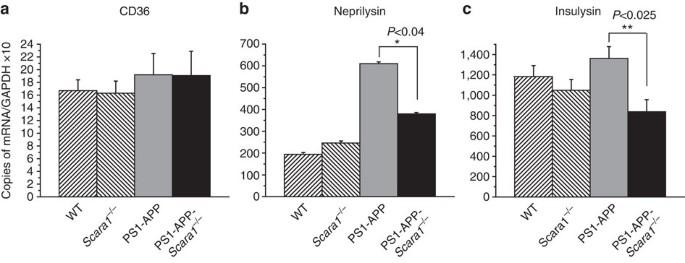Figure 5: Effect ofScara1deficiency on CD36 and Aβ-degrading enzymes. WT andScara1−/−mice express comparable mRNA levels of CD36 (a), and the Aβ-degrading enzymes neprilysin (b) and insulysin (c) in their brains. In contrast, PS1-APP-Scara1−/−mice express similar mRNA levels of CD36 as compared with PS1-APP mice (a), but significantly lower levels of neprilysin (b) and insulysin (c). Each bar is the average of three triplicate determinations per mouse from 3–5 different mice per genotype±s.e.m. (analysis of variance, *P<0.04, **P<0.025). GAPDH, glyceraldehyde 3-phosphate dehydrogenase. Figure 5: Effect of Scara1 deficiency on CD36 and Aβ-degrading enzymes. WT and Scara1 −/− mice express comparable mRNA levels of CD36 ( a ), and the Aβ-degrading enzymes neprilysin ( b ) and insulysin ( c ) in their brains. In contrast, PS1-APP- Scara1 − / − mice express similar mRNA levels of CD36 as compared with PS1-APP mice ( a ), but significantly lower levels of neprilysin ( b ) and insulysin ( c ). Each bar is the average of three triplicate determinations per mouse from 3–5 different mice per genotype±s.e.m. (analysis of variance, * P <0.04, ** P <0.025). GAPDH, glyceraldehyde 3-phosphate dehydrogenase. Full size image Aβ levels are also regulated by several Aβ-degrading enzymes such as neprilysin and insulysin [17] . To determine if increased Aβ levels in the brains of PS1-APP- Scara1 − / − mice are associated with reduced expression of neprilysin and/or insulysin, we measured mRNA levels of these two enzymes in the brains of young (150 days) WT, Scara1 −/− , PS1-APP and PS1-APP- Scara1 − / − mice. We found that expression of insulysin and neprilysin was comparable in WT and Scara1 − / − mice. Interestingly, expression of neprilysin was significantly higher in young PS1-APP mice compared with WT mice, suggesting that early in the disease process, uptake of Aβ may be associated with increased Aβ degradation. Expression of insulysin was also slightly higher in PS1-APP mice compared with WT mice, but the difference was small and did not reach statistical significance ( Fig. 5b ). In contrast, both neprilysin and insulin expression was significantly reduced by 38% and 36%, respectively, in PS1-APP- Scara1 − / − brains as compared with PS1-APP brains ( Fig. 5b ). These data suggest that phagocytosis of Aβ in young PS1-APP mice is associated with increased Aβ degradation, whereas decreased uptake of Aβ, as occurs in PS1-APP- Scara1 − / − mice, leads to decreased Aβ degradation and further increase in Aβ accumulation, thereby initiating a self-propagating loop of events that lead to accelerated disease progression. Data shown in Fig. 4a indicate that mortality of PS1-APP- Scara1 +/ − mice was only slightly better than that of PS1-APP- Scara1 − / − , but the difference did not reach statistical significance. To determine if partial Scara1 deficiency also affected AD-like pathology, we analysed the brains of young (150 days) PS1-APP- Scara1 +/ − mice for Aβ deposition in comparison with PS1-APP mice. As seen in Supplementary Fig. S3a , PS1-APP- Scara1 +/ − mice exhibited a significant increase in Aβ levels as measured by enzyme-linked immunosorbent assay (ELISA) (700 pg mg −1 brain protein versus 1500, pg mg −1 protein, P <0.002). This increase also correlated with increased visible Aβ deposits ( Supplementary Fig. S3b,c ). Of note, the number of visible Aβ deposits in ~150-day-old PS1-APP and PS1-APP- Scara1 +/− mice were small ( Supplementary Fig. S3b,c ), and we did not detect any Thioflavin S-positive deposits (not shown), suggesting that the majority of Aβ measured in these mice is in soluble or non-aggregated form. These data support the results obtained from our shRNA screen and from the experiments showing decreased uptake of sAβ in vitro by monocytes and microglia isolated from Scara1 -deficient mice. Upregulation of Scara1 leads to increased Aβ clearance Protollin, a proteosome-based adjuvant comprising purified outer-membrane proteins of Neisseria meningitides and lipopolysaccharide that is well tolerated in humans [23] , promotes increased accumulation of mononuclear phagocytes and increased clearance of amyloid when given intranasally to transgenic AD mice [24] , [25] . We investigated whether the mechanism by which Protollin enhances Aβ uptake by mononuclear phagocytes involves upregulation of Scara1 or CD36. As seen in Fig. 6a–c , although Protollin upregulated mRNA levels of Scara1 by more than threefold, it did not affect mRNA levels of CD36. Furthermore, Protollin upregulated Ccl2 mRNA levels by ~7 fold ( Fig. 6d ). These data suggest that the increased numbers of mononuclear phagocytes observed in Protollin-treated Alzheimer’s mice are may be because of their recruitment to sites of Aβ deposition via Ccl2. These data also suggest that Protollin-induced enhanced Aβ clearance may in part be due to increased recruitment of mononuclear phagocytes to Aβ-deposition sites. 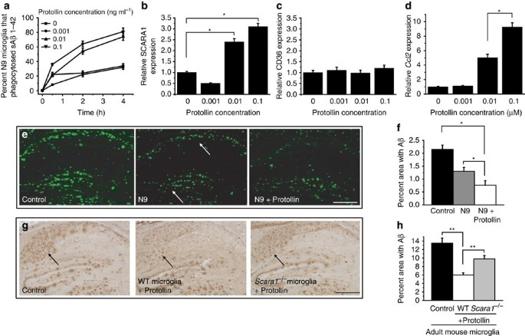Figure 6: Upregulation ofScara1increases sAβ uptakein vitroandin situin aScara1-dependent mechanism. (a) Protollin, a proteosome-based adjuvant comprising purified outer-membrane proteins ofN. meningitidesand lipopolysaccharide that is well tolerated in humans, upregulates sAβ uptake in N9 microglia. Cells were incubated for 18 h in presence of different concentrations of Protollin, and incubated with 0.5 μg ml−1sAβ 1–42, Hilyte-Fluor 488-labelled, for 30 min, 2 h and 4 h incubation. Cell-associated sAβ was measured by flow cytometry. (b,c) Protollin upregulatesScara1but not CD36 expression at the transcriptional level as measured by qPCR. (d) Protollin upregulates expression ofCcl2in a dose-dependent manner. N9 microglia were incubated with the indicated concentration of Protollin for 24 h, and expression ofScara1,CD36orCcl2was quantified by qPCR. (e,f) N9 microglia cells are plated on brain sections from a mouse model of AD for 24 h ±Protollin. The percent of the surface area of the brain covered by Aβ was measured by staining with anti-Aβ antibodies. (g,h) Reduction of amyloid load in the hippocampus following 24 h incubation with microglia isScara1dependent. Adult microglia isolated from WT andScara1−/−mice were added to brain sections from a mouse model of AD and incubated for 24 h ±Protollin. The percent of the surface area of the brain covered by Aβ was measured by staining with anti-Aβ antibodies. Scale bars, 500 μm. All data points represent the average of four independent determinations±s.e.m. (analysis of variance, *P<0.05, **P<0.03). Figure 6: Upregulation of Scara1 increases sAβ uptake in vitro and in situ in a Scara1 -dependent mechanism. ( a ) Protollin, a proteosome-based adjuvant comprising purified outer-membrane proteins of N. meningitides and lipopolysaccharide that is well tolerated in humans, upregulates sAβ uptake in N9 microglia. Cells were incubated for 18 h in presence of different concentrations of Protollin, and incubated with 0.5 μg ml −1 sAβ 1–42, Hilyte-Fluor 488-labelled, for 30 min, 2 h and 4 h incubation. Cell-associated sAβ was measured by flow cytometry. ( b , c ) Protollin upregulates Scara1 but not CD36 expression at the transcriptional level as measured by qPCR. ( d ) Protollin upregulates expression of Ccl2 in a dose-dependent manner. N9 microglia were incubated with the indicated concentration of Protollin for 24 h, and expression of Scara1 , CD36 or Ccl2 was quantified by qPCR. ( e , f ) N9 microglia cells are plated on brain sections from a mouse model of AD for 24 h ±Protollin. The percent of the surface area of the brain covered by Aβ was measured by staining with anti-Aβ antibodies. ( g , h ) Reduction of amyloid load in the hippocampus following 24 h incubation with microglia is Scara1 dependent. Adult microglia isolated from WT and Scara1 − / − mice were added to brain sections from a mouse model of AD and incubated for 24 h ±Protollin. The percent of the surface area of the brain covered by Aβ was measured by staining with anti-Aβ antibodies. Scale bars, 500 μm. All data points represent the average of four independent determinations±s.e.m. (analysis of variance, * P <0.05, ** P <0.03). Full size image Clearance of Aβ deposits in situ from brain sections derived from transgenic AD mice has been used as a surrogate measure for astrocyte ability to clear Aβ in vivo [26] . To test if Protollin-induced activation of N9 microglia promotes the ability of these cells to reduce Aβ deposits, we incubated these cells with brain sections derived from aged transgenic PS1-APP brains in the presence of increasing concentrations of Protollin. Such sections normally exhibit florid Aβ deposits in the cortex and hippocampus. As seen in Fig. 6e , the addition of Protollin-stimulated N9 microglia significantly reduced the size and number of Aβ deposits in such sections in the hippocampus when compared with untreated sections or sections incubated with unstimulated N9 microglia. To determine the relative importance of Scara1 in Aβ clearance by microglia activated with Protollin, we isolated WT and Scara1 − / − adult microglia as previously described [26] and compared their ability to clear brain Aβ deposits from PS1-APP brain slices as we did with N9 cells. After incubation of the brain sections with microglia from WT mice for 72 h, there was a 58% reduction in total Aβ deposits in the hippocampus ( P =0.0013) as compared with untreated sections and sections incubated with microglia from Scara1 − / − mice ( P =0.0214), which showed only a 20% reduction ( P =0.0317) as compared with untreated section ( Fig. 6g ). These data strongly support that Protollin-induced increased Aβ clearance is in part dependent on Scara1 and that pharmacological upregulation of Scara1 expression can be successfully accomplished. The role of mononuclear phagocytes including peripheral monocytes and microglia in AD is subject to intense investigation [27] . Although a shotgun approach that deletes all microglia for a brief period of time did not show an effect on amyloid deposition in a transgenic AD mouse model [28] , targeted genetic manipulation of the innate immune system in mouse models of AD provided strong evidence that mononuclear phagocytes have critical roles in regulating Aβ deposition by regulating the Aβ clearance pathways. Indeed, defects in microglial/mononuclear phagocyte accumulation in transgenic APP mice and other mouse models of AD are associated with increased Aβ deposition and increased mortality and/or cellular toxicity in these mice [1] , [29] . Furthermore, deficiencies and/or mutations in specific innate immune receptors such as CD14 and TLR4 affect Aβ deposition [30] , [31] . Unfortunately, with aging and progression of AD, innate immune cells of the brain appear to become dysfunctional, and their ability to clear amyloid becomes significantly reduced [4] . The exact mechanisms of such microglial dysfunction are not clear, but are believed to be at least, in part, due to downregulation of microglial Aβ phagocytic receptors [4] . In this manuscript, we provide direct evidence that the microglial/monocyte scavenger receptor Scara1 is a key Aβ clearance receptor expressed by these cells and that genetic deficiency in Scara1 is indeed associated with increased accumulation of Aβ. In addition, deficiency in Scara1 is associated with increased mortality in PS1-APP mice. Such increases in mortality and Aβ deposition are similar to what we observed in APP-Ccr2-deficient mice, and suggest that abnormalities in the number and/or function of mononuclear phagocytes can have detrimental effects on transgenic mouse models of AD. In contrast to the detrimental effects associated with dysfunction of the innate immune system in AD, we also show that restoring some of the Aβ-clearing ability of the innate immune system by pharmacological upregulation of Scara1 leads to increased Aβ clearance by mononuclear phagocytes and microglia, and therefore may be beneficial in slowing down or delaying progression of this disease. It is not clear if upregulating Scara1 expression by non-pharmacological approaches will also lead to increased sAβ clearance. Indeed, upregulating Scara1 mRNA in aging AD mice following irradiation does not seem to have the same effect as using Protollin [32] . It is possible that such apparent discrepancy may be due to increased influx of Aβ across the blood brain barrier as a result of increased permeability of the blood brain barrier following irradiation, to differences in the age and genotype of the mice analysed and/or the approach used to quantify sAβ. Nonetheless, our data clearly indicate that upregulating Scara1 expression pharmacologically is a viable therapeutic strategy to treat AD. We showed previously that blocking CD36-Aβ interactions reduces Aβ-induced activation of microglia to produce cytokines and reactive oxygen species [5] , [20] . We also showed that blocking these interactions does not affect phagocytosis of Aβ. Therefore, data from these papers indirectly support our findings in this manuscript that Scara1 , rather than CD36, is the main receptor for clearance of Aβ by mononuclear phagocytes. Our data also suggest that Scara1 and CD36 have complementary non-redundant roles in the interactions of mononuclear phagocytes with Aβ. Scara1 –Aβ interactions are beneficial and promote phagocytosis and clearance of Aβ, whereas CD36-Aβ interactions are harmful and lead to production of neurotoxins and pro-inflammatory molecules. This is reminiscent of the role that CD36 has in the interaction between macrophages and oxidized LDLs in atherosclerosis. Indeed, we have shown in the past that while Scara1 mediates adhesion to oxidized LDL-coated surfaces, CD36 mediates macrophage activation by oxidized LDL to produce reactive oxygen species [22] . In this regard, the findings presented in this manuscript draw an exciting, not yet described, parallel between atherosclerosis and AD. Dissecting the complex roles of various scavenger receptors in mononuclear phagocyte-Aβ interactions is therefore very important and, as we are showing in this manuscript, has therapeutic implications for AD. shRNA lentiviral infections Plasmids encoding lentiviruses expressing shRNAs were obtained from the RNAi Consortium library TRC-Mm1.0 (ref. 18 ), purified using the QiaPrep miniprep kit (Qiagen, Valencia, CA, USA) and then transfected into HEK 293T cells with a three-plasmid system to produce lentivirus. Infection conditions were optimized in 96-well plates. A total of 20,000 macrophages were placed in each well of 96-well tissue culture dishes and infected using 5 μl of shRNA lentiviral supernatant and 7.5 μg ml −1 polybrene. The cells were spun for 30 min at 2,000 r.p.m. and incubated for 24 h. To select for shRNA integration, infected cells were placed in puromycin (3 μg ml −1 ) and RPMI containing 10% fetal bovine serum (FBS). The cells were tested 1–2 weeks after infection. Mice PS1-APP bi-transgenic mice (B6C3-Tg (APPswe, PSEN1dE9)85Dbo/J stock number 004462) [33] , [34] were purchased from The Jackson Laboratories (Bar Harbor, ME, USA) and bred in the animal care facilities at Massachusetts General Hospital. Control mice are non-transgenic littermates of those PS1-APP mice expressing these transgenes. Scara1 − / − mice were generated by Professor Tatsuhiko Kodama, and a colony has been maintained in our lab for many years [35] . CD36 − / − mice were generated by Dr Kathryn Moore on a C57BL6 background, and a colony has been maintained in our lab for many years [5] . PS1-APP, Scara1 − / − and CD36 − / − mice were backcrossed for more than 13 generations on a C57BL/6 background. Lox-1 −/− mice [36] were a generous gift from Professor Tatsuya Sawamura, National Cardiovascular Center Research Institute Osaka, JAPAN. RAGE −/− mice [37] were a generous gift from Professor Hiroshi Yamamoto, Kanazawa, Japan. All protocols were approved by the Massachusetts General Hospital and Brigham and Women’s Hospital Institutional Animal Care and Use Committees and met the US National Institutes of Health guidelines for the humane care of animals. Stimulation and cell surface staining of N9 microglia N9 mouse microglia (a gift from Dr P. Riciarrdi-Castagnoli, University of Milano, Bicocca, Italy) [14] were plated on 24-well plates coated with 1 μg fibronectin per cm 2 (Sigma-Aldrich) and grown overnight in RPMI supplemented with10% FBS, L -glutamine (2 mM), penicillin 10 IU ml −1 and streptomycin 10 μg ml −1 . The following day, Protollin (GlaxoSmithKline, Laval, Quebec, Canada) was added and cells were incubated overnight. For staining, cells were lifted from the plate with CellStripper (Mediatech), resuspended in PBS/1% BSA/2% FBS containing 10 μg ml −1 Fc block (AbD Serotec) and then APC-labelled anti-mouse CD11b (1 μg ml −1 ) (BD Biosciences Pharmingen, San Diego, CA, USA), APC-labelled hamster anti-mouse CD36 clone HM36 (1 μg ml −1 ) (BioLegend, San Diego, CA, USA), Alexa647-labelled anti-CD204 (Scara1) clone 2F8 (2.5 μg ml −1 ) (AbD Serotec) or isotype-matched control antibodies (same concentrations as primary antibodies) were added and incubated on ice for 1 h. Cells were then fixed, and fluorescence intensity was measured using a FACScalibur (BD Biosciences) flow cytometer. Isolation of CD11b + microglia from adult brains Adult mouse microglia were isolated as described [4] . Briefly, 12-week-old mice were euthanized and perfused with 30cc PBS without Ca ++ and Mg ++ (PBS = ). Brains were then rinsed, minced and treated with Dispase and Collagenase Type 3 (Worthington Biochemicals, Lakewood, NJ, USA) for 45 min at 37 °C, followed by addition of 40 U ml −1 DNase I grade II (Roche Applied Science, Indianapolis, IN, USA) and incubation for an additional 15 min. The enzymes were inactivated by addition of 20 ml Hanks Balanced Salt Solution without Ca ++ and Mg ++ (HBSS = ) (Mediatech) containing 2 mM EDTA and 2% FBS, and the digested brain bits were triturated sequentially with a 25-, 10- and 5-ml pipette (8–10 times each step) and passed over a 100-μm filter (Fisher Scientific, Pittsburgh, PA, USA). Cells were centrifuged and resuspended in RPMI/ L -glutamine and mixed with physiological Percoll (Sigma-Aldrich), and centrifuged at 850 g for 45 min. The cell pellet was resuspended in RPMI, and the cells were passed over a 70-μm filter (Fisher Scientific), washed and then passed over a 40-μm filter (Fisher Scientific). The cells were then incubated with anti-mouse Cd11b-coated microbeads (Miltenyi Biotech, Auburn, CA, USA) and then washed. The bead-cell pellet was resuspended in PBS/0.5% BSA/2 mM EDTA and passed over a magnetic MACS Cell Separation column (Miltenyi Biotech) to separate Cd11b-positive cells (that is, cells that bound the beads—microglia/mononuclear phagocytes) from unbound Cd11b-negative cells (CD11b − ). Flow-through was collected and the column was rinsed 3 × with PBS/BSA/EDTA. CD11b-positive cells (CD11b + ) were eluted by removing the column from the magnetic holder and pushing PBS/BSA/EDTA through the column with a plunger. Cells were centrifuged and the pellets were resuspended in RPMI 1640 (Invitrogen) and used for experiments. Microglia isolated in this manner are more than 96% pure [4] . Isolation of monocytes from WT and knockout mice Monocytes were isolated by centrifugation over Ficoll 1077 as described for human monocytes [38] , [39] . This step removes neutrophils and red blood cells. The remaining cells include monocytes and lymphocytes. This was followed by adhesion to tissue culture plates for 1 h. The adherent cells (>90% monocytes) were then detached by brief incubation with 5 mM EDTA in PBS as described [38] . Quantitative real-time PCR Total RNA from each sample of cells (7.5–15 × 10 5 cells) was isolated using the RNeasy Plus mini kit (Qiagen) according to the manufacturer’s instructions and reverse transcribed using Multiscribe reverse transcriptase (Applied Biosystems, Foster City, CA, USA). Dilutions of each cDNA prep were used to assess β2-microglobulin RNA levels, and samples were then adjusted to give equivalent levels of β2-microglobulin per well in subsequent qPCR reactions for other genes. The qPCR was performed with the MX4000 unit (Agilent Technologies, Santa Clara, CA, USA) using SYBR Green to detect the amplification products as described [1] , [5] . The following cycles were performed: initial denaturation cycle 95 ° C for 10 min, followed by 40 amplification cycles of 95 ° C for 15 s and 60 ° C for 1 min, and ending with one cycle at 25 ° C for 15 s. Relative quantification of mRNA expression was calculated by the comparative cycle method described by the manufacturer (Agilent Technologies). For Scara1 qPCR, a standard curve for Scara1 was prepared from a plasmid (Open Biosystems, Huntsville, AL, USA) containing full-length mouse Scara1 , and then whole-brain RNA was isolated from triplicate samples using a Qiagen RNA easy Mini kit and quantified using a Thermo-Fisher Nanodrop (Waltham, MA). RNA of 1 μg was reverse transcribed into cDNA using Invitrogen’s First Strand Synthesis kit (Carlsbad, CA, USA), and qPCR was performed in a Roche 480 Lightcycler qPCR machine (Indianapolis, IN, USA) in triplicates for Scara1 (Forward primer: 5′-TGAACGAGAGGATGCTGACTG-3′, Reverse primer: 5′-GGAGGGGCCATTTTTAGTGC-3′) and compared with a standard curve of mouse Scara1 cDNA. Aβ ELISA For measurement of Aβ, we used commercially available ELISA kits (Invitrogen). Hemispheres of WT, PS1-APP and PS1-APP- Scara1 +/ − mice were homogenized in buffer containing 0.02 M guanidine and ELISA for Aβ performed according to the manufacturer’s instructions. In vitro uptake of Aβ by N9 cells N9 cells cultured in six-well plates were incubated overnight with various concentrations of Protollin. The cells were then incubated with PBS containing 1% BSA and 500 ng ml −1 Aβ 1–42 labelled with Alexa 488 (Anaspec, CA) for up to 4 h, then washed 3 × in PBS and lifted from the plate with CellStripper (Mediatech). Cells were then fixed by the addition of 2% paraformaldehyde. Cell-associated fluorescence intensity was measured using a FACScalibur (BD Biosciences) flow cytometer. Uptake of Aβ from brain sections and immunohistochemistry Brains from transgenic PS1-APP were collected and frozen unfixed in liquid nitrogen vapour and stored at −80 ° C, and 10–14-μm frozen sections were cut. N9 cells or WT microglia isolated from adult mice were then added in the presence of Protollin and incubated at 37 ° C for 24 h. Unbound cells were then rinsed in PBS, and the sections were fixed in 4% paraformaldehyde. To stain for Aβ, sections were blocked in PBS/0.3% Triton X-100/2% goat serum for 30 min, then incubated overnight at 25 ° C with rabbit anti-pan Aβ antibody (Biosource, Camarillo, CA, USA) or control antibody, at 2 μg ml −1 in PBS containing 0.3% Triton X-100 and 2% goat serum. The slides were then processed using the Vectastain Elite ABC Kit Rabbit IgG (Vector Laboratories, Burlingame, CA, USA) according to the manufacturer’s instructions. Vector NovaRed substrate kit for peroxidase (Vector Laboratories) was used to develop target-bound peroxidase for detection of Aβ in brain sections. Slides were counterstained with hematoxylin, mounted with VectaMount (Vector Laboratories), visualized by brightfield microscopy and digitally photographed. Alternatively, secondary anti rabbit IgG antibodies labelled with Alexa488 were used, and the slides were counterstained with 4′,6-diamidino-2-phenylindole, mounted using Vectashield (Vector Laboratories) and digitally photographed. For quantitation of the percent surface area stained with Anti-Aβ, five equally spaced sections were used per brain. Western blot of Scara1 Cell lysates of 2 μg were loaded onto a 10% SDS polyacrylamide gel (Invitrogen) transferred via iBlot (Invitrogen) onto polyvinylidene difluoride membrane, blocked for 1 h with 5% milk, then incubated with primary goat anti-mouse Scara1 antibodies (R&D Systems) followed by anti-goat horseradish peroxidase-labelled secondary antibody. The blots were then exposed to Hyperfilm (Amersham), developed and band intensity-quantified by densitometry with image J software. Statistical analysis Statistical analysis was performed using one-way analysis of variance with the Tukey’s test provided in the ‘Microcal Origin 8’ graphics and statistics software. P -values <0.05 where considered significant. How to cite this article: Frenkel, D. et al . Scara1 deficiency impairs clearance of soluble amyloid-β by mononuclear phagocytes and accelerates Alzheimer’s-like disease progression. Nat. Commun. 4:2030 doi: 10.1038/ncomms3030 (2013).